Lipid storage disorders block lysosomal trafficking by inhibiting a TRP channel and lysosomal calcium release Lysosomal lipid accumulation, defects in membrane trafficking and altered Ca 2+ homoeostasis are common features in many lysosomal storage diseases. Mucolipin transient receptor potential channel 1 (TRPML1) is the principle Ca 2+ channel in the lysosome. Here we show that TRPML1-mediated lysosomal Ca 2+ release, measured using a genetically encoded Ca 2+ indicator (GCaMP3) attached directly to TRPML1 and elicited by a potent membrane-permeable synthetic agonist, is dramatically reduced in Niemann–Pick (NP) disease cells. Sphingomyelins (SMs) are plasma membrane lipids that undergo sphingomyelinase (SMase)-mediated hydrolysis in the lysosomes of normal cells, but accumulate distinctively in lysosomes of NP cells. Patch-clamp analyses revealed that TRPML1 channel activity is inhibited by SMs, but potentiated by SMases. In NP-type C cells, increasing TRPML1's expression or activity was sufficient to correct the trafficking defects and reduce lysosome storage and cholesterol accumulation. We propose that abnormal accumulation of luminal lipids causes secondary lysosome storage by blocking TRPML1- and Ca 2+ -dependent lysosomal trafficking. The lysosome, which serves as the cell's recycling centre, can mediate the hydrolase-based degradation of a variety of biomaterials, including proteins, lipids and membranes [1] . Most lysosomal storage diseases (LSDs), of which more than 50 are known, are due to the defective activities of specific lysosomal enzymes, which result in the lysosomal accumulation of specific substrates [2] . For instance, in Niemann–Pick (NP) type A and B diseases (NPA and NPB), sphingomyelins (SMs) accumulate in lysosomes due to insufficient activity of acid SMase (aSMase) ( Supplementary Fig. S1 ) [3] ; similarly, insufficient aSMase activity and SM accumulation occur in NP type C (NPC), where the genetic defect occurs in components of an intracellular cholesterol/lipid trafficking pathway [3] , [4] . Interestingly, regardless of the nature of the primary undigested metabolites, common cellular defects are seen in a spectrum of LSDs [5] . For example, defects in lipid trafficking (the exit of lipids from the late endosome and lysosome) and autophagome–lysosome fusion are commonly observed in almost all sphingolipidoses, including NPA, NPB and NPC [2] , [6] . In addition, altered Ca 2+ and Fe 2+ homoeostasis are also common factors in these LSDs [2] , [5] , [7] . Thus, it is likely that the common trafficking machinery is impaired in LSDs with unrelated origins or primary defects. One intriguing hypothesis is that the primary accumulated materials cause a sort of 'lysosome stress,' which impairs common biochemical and/or signalling pathways in the lysosome, similar to the way unfolded proteins cause 'ER stress' to trigger an 'unfolded protein response' [2] , [5] . Cells that lack mucolipin transient receptor potential (TRP) channel 1 (TRPML1) exhibit lysosomal defects similar to those seen in NP cells: defective autophagosome–lysosome fusion or lysosome reformation, abnormal lipid trafficking and altered Ca 2+ and Fe 2+ homoeostasis [8] , [9] , [10] , [11] , [12] , [13] , [14] , [15] . Furthermore, mutations in the human Trpml1 gene cause mucolipidosis type IV (ML4) LSD, which exhibits membrane trafficking defects and excessive lysosomal storage [16] , [17] , [18] . TRPML1 is a ubiquitously expressed Fe 2+ and Ca 2+ dually permeable channel predominantly localized in late endosomes and lysosomes (LELs) [11] , [13] , [19] , [20] , [21] . TRPML1 is specifically activated by phosphatidylinositol 3,5-bisphosphate (PI(3,5)P 2 ), an LEL-localized low-abundance phosphoinositide [14] . In addition, both TRPML1-lacking and PI(3,5)P 2 -deficient cells exhibit defects in LEL-to-Golgi retrograde trafficking and autophagosome–lysosome fusion [8] , [15] , [22] , [23] , suggesting that the TRPML1-PI(3,5)P 2 system represents a common signalling pathway essential for late endocytic trafficking. Owing to the high degree of similarity in lysosomal defects, we hypothesized that TRPML1–PI(3,5)P 2 signalling is compromised in NPs and many other LSDs. In this study, we measured lysosomal Ca 2+ release with lysosome-targeted, genetically encoded Ca 2+ indicators and found that TRPML1-mediated lysosomal Ca 2+ release was compromised in NPC and NPA cells. Patch-clamp analyses demonstrated that TRPML1 channel activity was inhibited by micromolar concentrations of SMs, but potentiated by SM-hydrolysing enzyme SMases. In NPC cells, increasing TRPML1's expression or activity was found to be capable of correcting the trafficking defects and decrease cholesterol accumulation. We conclude that SMs are negative regulators of TRPML1 channels under physiological conditions, and that abnormal accumulation of SMs in the lysosome lumen blocks Ca 2+ -dependent membrane trafficking by directly inhibiting TRPML1. Identification of a potent synthetic agonist for TRPML1 A recent high-throughput screen identified 15 small-molecule chemical compounds (SF compounds) that can activate recombinant surface-expressed TRPML3 [21] . TRPML1 is primarily localized on the membranes of LELs [13] . Using whole-endolysosome patch-clamp recordings [11] , [14] , we found that several SF compounds also weakly activated whole-endolysosome TRPML1-mediated currents ( I TRPML1 or I ML1 , data not shown). In HEK293T cells transfected with surface-expressed mutant TRPML1 channels (TRPML1-L 15 L/AA-L 577 L/AA, abbreviated as ML1-4A [9] , [21] ), one of the SF compounds, SF-51 [21] , induced small cytosolic Ca 2+ ([Ca 2+ ] cyt ) increases (measured with Fura-2 ratios; Fig. 1a,b ), and activated small but significant inwardly rectifying whole-cell currents ( I ML1−4A ; Fig. 1d ). 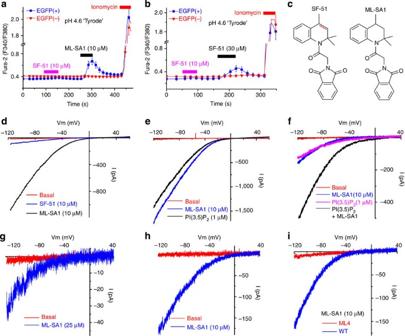Figure 1: Activation of TRPML1 by small-molecule synthetic agonists. (a) ML-SA1 induced increases in cytosolic [Ca2+], as measured by the Fura-2 ratio (F340/F380) in HEK293T cells expressing TRPML1-L15L/AA-L577L/AA (ML1-4A) at low pH (pH 4.6) external solution. SF-51 (10 μM) induced much smaller responses in the same cells. (b) SF-51 (30 μM) induced increases in cytosolic [Ca2+] in ML1-4A-expressing HEK293T cells at low pH external solution. (c) Chemical structures of SF-51 and ML-SA1. The difference between SF-51 and ML-SA1 is highlighted in red. (d) Activation of whole-cell currents by SF-51 and ML-SA1 in ML1-4A-expressing HEK293T cells. ML1-4A-mediated current (IML1−4A) was elicited by repeated voltage ramps (−140 to +140 mV; 400 ms) with a 4-s interval between ramps. Only a portion of the voltage protocol is shown; holding potential=0 mV. (e) Activation of whole-endolysosomeIML1by ML-SA1 and PI(3,5)P2. Enlarged vacuoles/endolysosomes were isolated from vacuolin-treated HEK293 cells stably expressing ML1-4A. ML-SA1 and PI(3,5)P2were applied to the cytosolic sides of the isolated vacuoles. The pipette (luminal) solution was a standard external (Tyrode's) solution adjusted to pH 4.6; the bath (internal/cytoplasmic) solution was a K+-based solution (140 mM K+-gluconate). Note that the inward current indicates cations flowing out of the endolysosome. (f) Synergistic activation of whole-endolysosomeIML1by ML-SA1 and PI(3,5)P2in human fibroblasts.IML1was activated by PI(3,5)P2(1 μM) and ML-SA1 (10 μM); coapplication of PI(3,5)P2and ML-SA1 further increasedIML1. (g) ML-SA1 activated endogenous whole-endolysosome ML-like currents (IML−L) in CHO cells. (h) ML-SA1 activated whole-endolysosomeIML−Lin mouse primary macrophages. (i) ML-SA1 activated whole-endolysosomeIML1in WT (ML1+/+), but not ML4 (ML1−/−), human fibroblasts. For panels a and b, the responses were averaged for 20–40 cells from one representative experiment; dara are presented as the mean±s.e.m. Figure 1: Activation of TRPML1 by small-molecule synthetic agonists. ( a ) ML-SA1 induced increases in cytosolic [Ca 2+ ], as measured by the Fura-2 ratio ( F 340 / F 380 ) in HEK293T cells expressing TRPML1-L 15 L/AA-L 577 L/AA (ML1-4A) at low pH (pH 4.6) external solution. SF-51 (10 μM) induced much smaller responses in the same cells. ( b ) SF-51 (30 μM) induced increases in cytosolic [Ca 2+ ] in ML1-4A-expressing HEK293T cells at low pH external solution. ( c ) Chemical structures of SF-51 and ML-SA1. The difference between SF-51 and ML-SA1 is highlighted in red. ( d ) Activation of whole-cell currents by SF-51 and ML-SA1 in ML1-4A-expressing HEK293T cells. ML1-4A-mediated current ( I ML1−4A ) was elicited by repeated voltage ramps (−140 to +140 mV; 400 ms) with a 4-s interval between ramps. Only a portion of the voltage protocol is shown; holding potential=0 mV. ( e ) Activation of whole-endolysosome I ML1 by ML-SA1 and PI(3,5)P 2 . Enlarged vacuoles/endolysosomes were isolated from vacuolin-treated HEK293 cells stably expressing ML1-4A. ML-SA1 and PI(3,5)P 2 were applied to the cytosolic sides of the isolated vacuoles. The pipette (luminal) solution was a standard external (Tyrode's) solution adjusted to pH 4.6; the bath (internal/cytoplasmic) solution was a K + -based solution (140 mM K + -gluconate). Note that the inward current indicates cations flowing out of the endolysosome. ( f ) Synergistic activation of whole-endolysosome I ML1 by ML-SA1 and PI(3,5)P 2 in human fibroblasts. I ML1 was activated by PI(3,5)P 2 (1 μM) and ML-SA1 (10 μM); coapplication of PI(3,5)P 2 and ML-SA1 further increased I ML1 . ( g ) ML-SA1 activated endogenous whole-endolysosome ML-like currents ( I ML−L ) in CHO cells. ( h ) ML-SA1 activated whole-endolysosome I ML−L in mouse primary macrophages. ( i ) ML-SA1 activated whole-endolysosome I ML1 in WT (ML1 +/+ ), but not ML4 (ML1 −/− ), human fibroblasts. For panels a and b, the responses were averaged for 20–40 cells from one representative experiment; dara are presented as the mean±s.e.m. Full size image By conducting a Fura-2-based low-throughput screen for more potent TRPML1 agonists, we identified a SF-51-related compound ( Fig. 1c for the chemical structures; Mucolipin Synthetic Agonist 1 or ML-SA1) that could induce significant [Ca 2+ ] cyt increases in HEK293 cells stably or transiently expressing ML1-4A ( Fig. 1a ). In electrophysiological assays, ML-SA1 robustly activated whole-cell I ML1−4A ( Fig. 1d ) and whole-endolysosome I ML1 ( Fig. 1e ). ML-SA1 also activated whole-cell I TRPML2 and I TRPML3 , but not six other related channels ( Supplementary Fig. S2 ). ML-SA1 (10 μM) activation of whole-endolysosome I ML1 was comparable to the effect of the endogenous TRPML agonist PI(3,5)P 2 (1 μM; Fig. 1e ), and these agonists were synergistic with each other ( Fig. 1f ). ML-SA1 activated an endogenous whole-endolysosome TRPML-like current ( I ML−L ) in all mammalian cell types that we investigated, including Chinese Hamster Ovary (CHO) ( Fig. 1g ), Cos-1, HEK293, skeletal muscle, pancreatic β and macrophage cells ( Fig. 1h ). ML-SA1 activated whole-endolysosome I ML−L in wild-type (WT; ML1 +/+ ), but not ML4 (ML1 −/− ) human fibroblasts ( Fig. 1i ), suggesting that although ML-SA1 targets all three TRPMLs, the expression levels of TRPML2 and TRPML3 are very low, and TRPML1 is the predominant lysosomal TRPML channel in this cell type. Thus, we have identified a reasonably specific and potent agonist that can be a useful chemical tool for studying the functions of TRPMLs, especially TRPML1. A lysosome-targeted genetically encoded Ca 2+ indicator To measure lysosomal Ca 2+ release in intact cells, we engineered GCaMP3, a single-wavelength genetically encoded Ca 2+ indicator [24] , to the cytoplasmic amino terminus of TRPML1 ( Fig. 2a ). When transfected into HEK293T, CHO or Cos-1 cell lines, GCaMP3-TRPML1 (GCaMP3-ML1) was mainly localized in the Lamp-1 and LysoTracker-positive compartments, that is, LEL ( Fig. 2b,c ). To determine the specificity of the GCaMP3-ML1 fluorescence signal, we tested a variety of Ca 2+ release reagents and found that GCaMP3 fluorescence ( F 470 ) responded preferentially and reliably to lysosome-acting Ca 2+ -mobilization reagents (Δ F / F 0 =0.2–1), including glycyl- L -phenylalanine 2-naphthylamide (GPN, a Cathepsin C substrate that induces osmotic lysis of lysosomes; Fig. 2d ) and bafilomycin A1 (Baf-A1, a V-ATPase inhibitor) [25] . In a subset of cells, GCaMP3 also responded to large (Δ F / F 0 >2) Ca 2+ increases triggered by thapsigargin (targeting the endoplasmic recticulum (ER) Ca 2+ store; Fig. 2d ), which may presumably spread to close proximity of lysosomes. In the majority of the cells, however, TG failed to significantly increase GCaMP3 fluorescence ( Fig. 2d ), suggesting that small ER Ca 2+ release was not detected by GCaMP3-ML1. Taken together, GCaMP3-ML1 readily and preferentially detects juxta-lysosomal Ca 2+ increases. 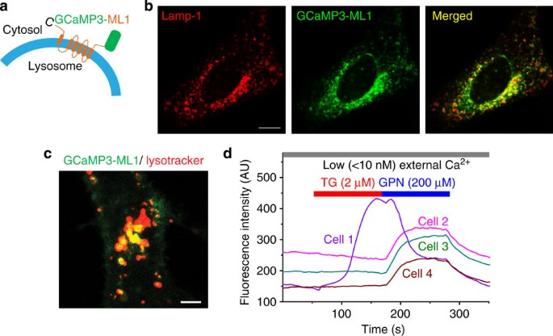Figure 2: A lysosome-targeted genetically encoded Ca2+indicator. (a) GCaMP3–TRPML1 (GCaMP3–ML1) fusion strategy. GCaMP3 is fused to the N-terminus of TRPML1. (b) Colocalization of GCaMP3-ML1 fluorescence with Lamp-1 in HEK293T cells expressing both GCaMP3-ML1 and Lamp-1-mCherry. Scale bar=5 μm. (c) Colocalization of GCaMP3-ML1 fluorescence with LysoTracker in GCaMP3-ML1-expressing HEK293T cells. Scale bar=2 μm. (d) Preferential detection of Ca2+release from lysosome stores by GCaMP3-ML1 in GCaMP3-ML1-transfected Cos-1 cells. ER and lysosome Ca2+releases were triggered by thapsigargin (TG, 2 μM) and GPN (200 μM), respectively, in low (nominally free Ca2++ 1 mM EGTA; free [Ca2+] estimated to be <10 nM) external [Ca2+]. All cells responded to GPN; only one out of four cells responded to TG. Figure 2: A lysosome-targeted genetically encoded Ca 2+ indicator. ( a ) GCaMP3–TRPML1 (GCaMP3–ML1) fusion strategy. GCaMP3 is fused to the N-terminus of TRPML1. ( b ) Colocalization of GCaMP3-ML1 fluorescence with Lamp-1 in HEK293T cells expressing both GCaMP3-ML1 and Lamp-1-mCherry. Scale bar=5 μm. ( c ) Colocalization of GCaMP3-ML1 fluorescence with LysoTracker in GCaMP3-ML1-expressing HEK293T cells. Scale bar=2 μm. ( d ) Preferential detection of Ca 2+ release from lysosome stores by GCaMP3-ML1 in GCaMP3-ML1-transfected Cos-1 cells. ER and lysosome Ca 2+ releases were triggered by thapsigargin (TG, 2 μM) and GPN (200 μM), respectively, in low (nominally free Ca 2+ + 1 mM EGTA; free [Ca 2+ ] estimated to be <10 nM) external [Ca 2+ ]. All cells responded to GPN; only one out of four cells responded to TG. Full size image In GCaMP3-ML1-transfected CHO ( Fig. 3a,b ), HEK293T and Cos-1 cell lines, application of ML-SA1 (20 μM) induced rapid increases in GCaMP3 fluorescence (Δ F / F 0 =0.45±0.05, n =77 cells; Fig. 3a,k ) in the presence of low external Ca 2+ (nominally free Ca 2+ + 1 mM EGTA; free Ca 2+ estimated to be <10 nM). By contrast, no significant increase in GCaMP3 fluorescence (Δ F / F 0 =0.03±0.01, n =32 cells; Fig. 3c,d and k ) was observed in cells transfected with a plasmid carrying GCaMP3 fused to a non-conducting pore mutant of TRPML1 [8] , [14] (GCaMP3-ML1-KK). Both GPN and Baf-A1 largely abolished ML-SA1-induced Ca 2+ responses ( Fig. 3e–k ). By contrast, ML-SA1-induced Ca 2+ response was mostly intact in TG-treated cells ( Fig. 3k ). Collectively, these results suggest that ML-SA1 activated endolysosomal TRPML1 to induce Ca 2+ release from lysosomes. Thus, we have established a robust Ca 2+ imaging assay to measure TRPML1-mediated lysosomal Ca 2+ release. 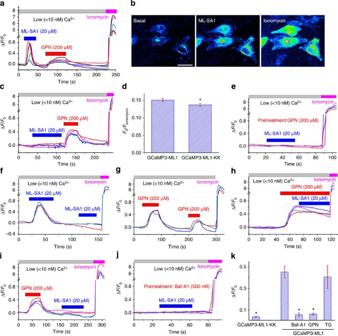Figure 3: ML-SA1 induces TRPML1-mediated Ca2+release from lysosomes. (a) ML-SA1 (20 μM) induced rapid increases in GCaMP3 fluorescence (measured as change of GCaMP3 fluorescence ΔFover basal fluorescenceF0; ΔF/F0) under low (< 10 nM) external Ca2+in CHO cells transfected with GCaMP3-ML1. Subsequent application of GPN (200 μM) induced smaller responses. Maximal responses were induced by ionomycin (1 μM) application. (b) Representative micrographs from panel (a) to show the changes of GCaMP3 fluorescence upon bath application of ML-SA1 and ionomycin to GCaMP3-ML1-transfected CHO cells. Scale bar=5 μm. (c) ML-SA1 failed to induce significant Ca2+increases in CHO cells transfected with GCaMP3-ML1-KK (non-conducting pore mutation). (d) Basal GCaMP3 fluorescence (normalized to the maximal ionomycin-induced fluorescence) of GCaMP3-ML1-KK and GCaMP3-ML1. (e) GPN (200 μM) pretreatment abolished ML-SA1-induced responses in GCaMP3-ML1-expressing CHO cells. (f) Repetitive applications of ML-SA1 (20 μM) induced little or no responses in GCaMP3-ML1-expressing CHO cells. (g) Repetitive applications of GPN (200 μM) induced smaller GCaMP3 responses in GCaMP3-ML1-expressing CHO cells. (h) ML-SA1 failed to further increase GCaMP3 fluorescence in GCaMP3-ML1-expressing CHO cells in the presence of GPN (200 μM). (i) ML-SA1 induced small responses in GCaMP3-ML1-expressing CHO cells that had received an application of GPN. (j) Baf-A1 (500 nM) pretreatment abolished ML-SA1-induced Ca2+response in GCaMP3-ML1-expressing CHO cells. (k) ML-SA1-induced responses in CHO cells transfected with GCaMP3-ML1-KK (non-conducting pore mutation), and GCaMP3-ML1-transfected cells pretreated with Baf-A1, GPN or TG. For panelsdandk, the responses were averaged for 40–100 transfected cells from at least three independent experiments; data are presented as the mean±s.e.m. Statistical comparisons were made using analysis of variance: *P<0.05. Figure 3: ML-SA1 induces TRPML1-mediated Ca 2+ release from lysosomes. ( a ) ML-SA1 (20 μM) induced rapid increases in GCaMP3 fluorescence (measured as change of GCaMP3 fluorescence Δ F over basal fluorescence F 0 ; Δ F / F 0 ) under low (< 10 nM) external Ca 2+ in CHO cells transfected with GCaMP3-ML1. Subsequent application of GPN (200 μM) induced smaller responses. Maximal responses were induced by ionomycin (1 μM) application. ( b ) Representative micrographs from panel ( a ) to show the changes of GCaMP3 fluorescence upon bath application of ML-SA1 and ionomycin to GCaMP3-ML1-transfected CHO cells. Scale bar=5 μm. ( c ) ML-SA1 failed to induce significant Ca 2+ increases in CHO cells transfected with GCaMP3-ML1-KK (non-conducting pore mutation). ( d ) Basal GCaMP3 fluorescence (normalized to the maximal ionomycin-induced fluorescence) of GCaMP3-ML1-KK and GCaMP3-ML1. ( e ) GPN (200 μM) pretreatment abolished ML-SA1-induced responses in GCaMP3-ML1-expressing CHO cells. ( f ) Repetitive applications of ML-SA1 (20 μM) induced little or no responses in GCaMP3-ML1-expressing CHO cells. ( g ) Repetitive applications of GPN (200 μM) induced smaller GCaMP3 responses in GCaMP3-ML1-expressing CHO cells. ( h ) ML-SA1 failed to further increase GCaMP3 fluorescence in GCaMP3-ML1-expressing CHO cells in the presence of GPN (200 μM). ( i ) ML-SA1 induced small responses in GCaMP3-ML1-expressing CHO cells that had received an application of GPN. ( j ) Baf-A1 (500 nM) pretreatment abolished ML-SA1-induced Ca 2+ response in GCaMP3-ML1-expressing CHO cells. ( k ) ML-SA1-induced responses in CHO cells transfected with GCaMP3-ML1-KK (non-conducting pore mutation), and GCaMP3-ML1-transfected cells pretreated with Baf-A1, GPN or TG. For panels d and k , the responses were averaged for 40–100 transfected cells from at least three independent experiments; data are presented as the mean±s.e.m. Statistical comparisons were made using analysis of variance: * P <0.05. Full size image Reduced TRPML1-mediated lysosomal Ca 2+ release in NPC cells Next, we investigated whether TRPML1-mediated lysosomal Ca 2+ release is altered in NP cells. We chose an easy-to-transfect cellular model of NPC, NPC (NPC1 −/− ) CHO cells, which exhibit all the hallmark features of NPC disease [26] , [27] . WT CHO cells transfected with GCaMP3-ML1 exhibited large TRPML1-mediated lysosomal Ca 2+ release ( Fig. 4a,l ). In contrast, NPC CHO cells exhibited much smaller TRPML1-mediated Ca 2+ release with a ~75% reduction compared with WT controls ( Fig. 4b,l ). GCaMP3-ML1 was still mainly colocalized with Lamp-1 in NPC cells ( Fig. 4c ). In addition, the expression levels of GCaMP3-ML1, as estimated from the maximal fluorescence intensity induced by ionomycin, were comparable for WT and NPC cells ( Fig. 4d ). A previous study reported that lysosomal Ca 2+ stores are compromised in NPC cells [25] . However, we found that GPN-induced GCaMP3-ML1 increases were comparable for WT and NPC cells ( Fig. 4e ). Likewise, GPN-induced and NH 4 Cl-induced Fura-2 responses were also comparable in non-transfected WT and NPC cells ( Fig. 4f,g ). Furthermore, TRPML1-mediated, but not GPN-induced lysosomal Ca 2+ release, was also reduced in GCaMP3-transfected NPC human fibroblasts compared with WT cells ( Fig. 4h ). Collectively, these results suggest that TRPML1-mediated lysosomal Ca 2+ release is selectively reduced in NPC cells. 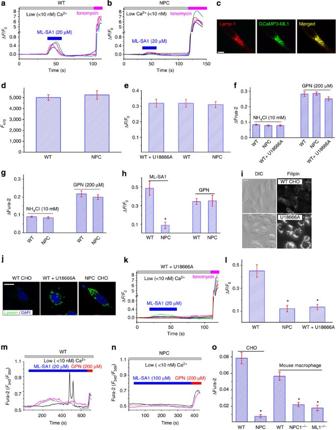Figure 4: Lysosomal Ca2+release via TRPML1 is reduced in NPC cells. (a,b) ML-SA1-induced lysosomal Ca2+release in GCaMP3-ML1-transfected WT (a) and NPC (b) CHO cells. (c) Colocalization of GCaMP3-ML1 fluorescence with Lamp-1 in NPC CHO cells doubly transfected with GCaMP3-ML1 and Lamp-1-mCherry. Scale bar=5 μm. (d) Comparable expression levels of GCaMP3-ML1 in WT and NPC CHO cells. Expression level of GCaMP3-ML1 was estimated by the maximal GCaMP3 fluorescence signal induced by ionomycin (1 μM). (e) Comparable GPN-induced GCaMP3 responses in WT, NPC or U18666A-treated GCaMP3-ML1-transfected CHO cells. (f) NH4Cl (10 mM) and GPN (200 μM) induced comparable levels of Ca2+increases (measured with Fura-2 ratios) in WT, NPC and U18666A-treated CHO cells. (g) NH4Cl (10 mM) and GPN (200 μM) induced comparable levels of Fura-2 Ca2+responses in WT and NPC human fibroblasts. (h) TRPML1-mediated, but not GPN-induced, lysosomal Ca2+release was reduced in GCaMP3-ML1-transfected NPC human fibroblasts compared with WT cells. (i) WT CHO cells were treated with U18666A (2 μg ml−1) for 16 h, and then subjected to filipin staining. Scale bar=10 μm. (j) SMs were stained with Lysenin (0.1 μg ml−1) in WT CHO cells, WT CHO cells treated with U18666A (2 μg ml−1) for 16 h and NPC CHO cells. Scale bar=10 μm. (k) Ca2+responses in GCaMP3-ML1-transfected WT CHO cells treated with U18666A (2 μg ml−1) for 16–20 h. (l) ML-SA1-induced peak GCaMP3 responses were reduced in GCaMP3-ML1-transfected NPC or U18666A-treated WT CHO cells. (m,n) Endogenous TRPML1-mediated lysosomal Ca2+release (measured with Fura-2 ratios) in WT (m) and NPC (n) CHO cells. (o) Average endogenous ML-SA1-induced lysosomal Ca2+responses in WT and NPC CHO cells, and WT, NPC1−/−and ML1−/−mouse macrophages. For panelsd,e,f,g,h,k,lando, the results were averaged for 40–100 cells from at least three independent experiments; data are presented as the mean±s.e.m. Statistical comparisons were made using analysis of variance: *P<0.05. Figure 4: Lysosomal Ca 2+ release via TRPML1 is reduced in NPC cells. ( a , b ) ML-SA1-induced lysosomal Ca 2+ release in GCaMP3-ML1-transfected WT ( a ) and NPC ( b ) CHO cells. ( c ) Colocalization of GCaMP3-ML1 fluorescence with Lamp-1 in NPC CHO cells doubly transfected with GCaMP3-ML1 and Lamp-1-mCherry. Scale bar=5 μm. ( d ) Comparable expression levels of GCaMP3-ML1 in WT and NPC CHO cells. Expression level of GCaMP3-ML1 was estimated by the maximal GCaMP3 fluorescence signal induced by ionomycin (1 μM). ( e ) Comparable GPN-induced GCaMP3 responses in WT, NPC or U18666A-treated GCaMP3-ML1-transfected CHO cells. ( f ) NH 4 Cl (10 mM) and GPN (200 μM) induced comparable levels of Ca 2+ increases (measured with Fura-2 ratios) in WT, NPC and U18666A-treated CHO cells. ( g ) NH 4 Cl (10 mM) and GPN (200 μM) induced comparable levels of Fura-2 Ca 2+ responses in WT and NPC human fibroblasts. ( h ) TRPML1-mediated, but not GPN-induced, lysosomal Ca 2+ release was reduced in GCaMP3-ML1-transfected NPC human fibroblasts compared with WT cells. ( i ) WT CHO cells were treated with U18666A (2 μg ml −1 ) for 16 h, and then subjected to filipin staining. Scale bar=10 μm. ( j ) SMs were stained with Lysenin (0.1 μg ml −1 ) in WT CHO cells, WT CHO cells treated with U18666A (2 μg ml −1 ) for 16 h and NPC CHO cells. Scale bar=10 μm. ( k ) Ca 2+ responses in GCaMP3-ML1-transfected WT CHO cells treated with U18666A (2 μg ml −1 ) for 16–20 h. ( l ) ML-SA1-induced peak GCaMP3 responses were reduced in GCaMP3-ML1-transfected NPC or U18666A-treated WT CHO cells. ( m , n ) Endogenous TRPML1-mediated lysosomal Ca 2+ release (measured with Fura-2 ratios) in WT ( m ) and NPC ( n ) CHO cells. ( o ) Average endogenous ML-SA1-induced lysosomal Ca 2+ responses in WT and NPC CHO cells, and WT, NPC1 −/− and ML1 −/− mouse macrophages. For panels d , e , f , g , h , k , l and o , the results were averaged for 40–100 cells from at least three independent experiments; data are presented as the mean±s.e.m. Statistical comparisons were made using analysis of variance: * P <0.05. Full size image NPC-like cellular phenotypes can be pharmacologically induced with a small-molecule drug U18666A [28] . After incubating GCaMP3-ML1-transfected WT CHO cells with U18666A (2 μg ml −1 ) for 16–20 h, cells exhibited significant increases in cholesterol level as detected by filipin staining [4] ( Fig. 4i ), and sphingomyelin (SM) level as detected by lysenin staining ( Fig. 4j ). U18666A-treated cells exhibited a ~70% reduction in TRPML1-mediated lysosomal Ca 2+ release ( Fig. 4k,l ). Conversely, drug treatment failed to result in noticeable changes in GPN-induced GCaMP3 responses ( Fig. 4e ) or Fura-2 Ca 2+ responses ( Fig. 4f ). Taken together, these results suggest a specific reduction of TRPML1-mediated lysosomal Ca 2+ release in pharmacologically induced NPC cells. We next investigated the effect of NPC on endogenous Ca 2+ release using Fura-2 Ca 2+ imaging. In WT CHO cells, small but significant Ca 2+ increases were seen upon application of 100 μM ML-SA1 in low external Ca 2+ (ΔFura-2=0.08±0.01, n =89; Fig. 4m,o ). In contrast, in NPC CHO cells, ML-SA1 failed to induce significant Ca 2+ responses (ΔFura-2=0.01±0.002, n =61; Fig. 4n,o ). Cyclodextrin, a polysaccharide that reportedly alleviates NPC cellular phenotypes [4] , was found to partially restore ML-SA1-induced lysosomal Ca 2+ release ( Supplementary Fig. S3 ). Finally, NPC1 −/− mouse macrophages, one of the major cell types affected in NPC [3] , also exhibited a significant reduction in ML-SA1-induced lysosomal Ca 2+ release compared with WT cells ( Fig. 4o and Supplementary Fig. S4 ). The ML-SA1-induced lysosomal Ca 2+ responses are most likely mediated by TRPML1, as demonstrated by the lack of response in ML1 −/− macrophages ( Fig. 4o and Supplementary Fig. S4 ). Collectively, the reduction in TRPML1-mediated lysosomal Ca 2+ release may be a general feature of most NPC cell types. Reduced TRPML1-mediated currents in NPC cell lysosomes We next investigated the effect of NPC on whole-endolysosome I ML1 in human fibroblasts. Compared with WT fibroblasts ( Fig. 5a,c ), much smaller ML-SA1-activated I ML1 was seen in NPC fibroblasts at three different concentrations of ML-SA1 ( Fig, 5b,c ). On average, whole-endolysosome I ML1 activated by 25 μM ML-SA1 was 75±25 pA/pF ( n =8) for NPC cells, a ~70% reduction from the values observed for WT cells (442±150 pA/pF; n =6). Notably, the messenger RNA expression levels of TRPML1-3 were not decreased in NPC cells ( Fig, 5d ). These results suggest that a reduction of whole-endolysosome I ML1 accounts for the reduced TRPML1-mediated Ca 2+ release observed in NPC cells. 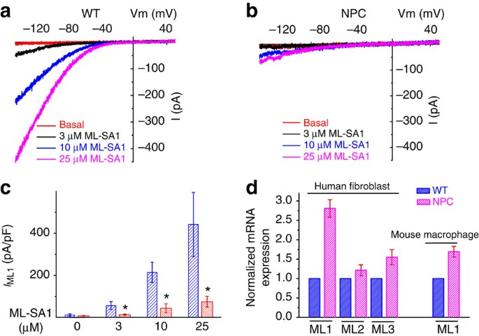Figure 5: TRPML-mediated currents are reduced in the lysosomes of NPC cells. (a,b) Concentration-dependent activation of whole-endolysosomeIML−Lin WT (a) and NPC (b) human fibroblasts. ML-SA1 (3, 10 and 25 μM) was applied to the cytosolic sides of the vacuoles isolated from human fibroblasts. (c) Average current densities (pA/pF) ofIML−Lwere reduced in NPC fibroblasts compared with WT cells. The current density was calculated from the current size (pA) normalized with the capacitance of the vacuole (pF). (d) Reverse transcriptase PCR analysis ofTRPML1-3messenger RNA expression in WT and NPC human fibroblasts, and NPC1−/−mouse macrophages. Expression levels were normalized to that of glyceraldehyde-3-phosphate dehydrogenase (human fibroblast) and L32 (mouse macrophage). For panelscandd, data are presented as the mean±s.e.m. (WT (blue),n=6; NPC (red),n=8). Statistical comparisons were made using analysis of variance: *P<0.05. Figure 5: TRPML-mediated currents are reduced in the lysosomes of NPC cells. ( a , b ) Concentration-dependent activation of whole-endolysosome I ML−L in WT ( a ) and NPC ( b ) human fibroblasts. ML-SA1 (3, 10 and 25 μM) was applied to the cytosolic sides of the vacuoles isolated from human fibroblasts. ( c ) Average current densities (pA/pF) of I ML−L were reduced in NPC fibroblasts compared with WT cells. The current density was calculated from the current size (pA) normalized with the capacitance of the vacuole (pF). ( d ) Reverse transcriptase PCR analysis of TRPML1-3 messenger RNA expression in WT and NPC human fibroblasts, and NPC1 −/− mouse macrophages. Expression levels were normalized to that of glyceraldehyde-3-phosphate dehydrogenase (human fibroblast) and L32 (mouse macrophage). For panels c and d , data are presented as the mean±s.e.m. (WT (blue), n =6; NPC (red), n =8). Statistical comparisons were made using analysis of variance: * P <0.05. Full size image Inhibition of TRPML1 by SMs The reduced TRPML1-mediated lysosomal Ca 2+ release and I ML1 in the presence of normal TRPML1 expression in NPC cells suggest tonic inhibition of TRPML1 by cytoplasmic and/or luminal factors. One possibility is that lipids accumulated in NPC lysosomes, such as cholesterol, SM, sphingosine and glycosphingolipids [4] , [29] , might directly inhibit TRPML1. To test this possibility, we performed whole-cell recordings in ML1-4A-expressing HEK293T cells. Under this configuration, the extracellular side is analogous to the luminal side ( Supplementary Fig. S1 ), making it possible to study the effects of luminal lipids on I ML1−4A . SMs, but not cholesterol or glycosphingolipids (data not shown), acutely inhibited SF-51- ( Fig, 6a,d ) or ML-SA1-activated I ML1−4A . In contrast, SMs failed to inhibit I ML1−Va, a gain-of-function mutation that locks TRPML1 in the open state [13] ( Fig. 6b,d ). SMs can be hydrolysed into ceramide and phosphocholine by SMase ( Supplementary Fig. S1 ). No significant inhibition was seen with ceramide ( Fig. 6c,d ) or phosphocholine ( Fig. 6d ). Sphingosine, a hydrolysed product of ceramide, potentiated I ML1−4A ( Fig. 6e ). 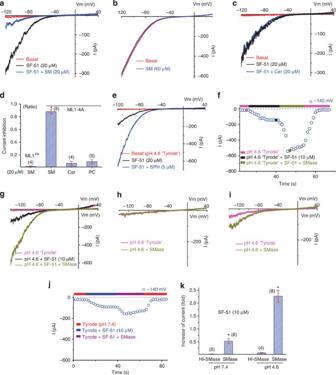Figure 6: Regulation of TRPML1 by SMs and sphingomyelinases. (a) SF-51-activated whole-cellIML1−4Awas inhibited by SMs (20 μM) at low extracellular pH in ML1-4A-expressing HEK293T cells. (b) Insensitivity of whole-cellIML1−Vato SMs (60 μM). (c) Lack of effect of ceramide (Cer, 20 μM) on whole-cellIML1−4A. (d) Summary of the effects of various sphingolipids on whole-cellIML1−4Ain ML1-4A-expressing HEK293T cells. PC: phosphocholine. (e) SF-51-activated whole-cellIML1−4Awas potentiated by sphingosine (Sph; 5 μM) at low external pH in ML1-4A-expressing HEK293T cells. (f) The effects of SMase (50 ng ml−1) treatment onIML1−4Aat low external pH.IML1−4Awas elicited by repeated voltage ramps (−140 to + 140 mV; 400 ms) with a 4-s interval between ramps. Current amplitudes at −140 mV were used to plot the time dependence. (g) Representative traces ofIML1−4Abefore (black) and after (dark yellow) SMase treatment at two different time points, as shown inf. (h,i) SMase (50 ng ml−1) treatment alone had no (six out of seven cells; seehfor an example) or small (one out of seven cells;i) activation effect on basal whole-cellIML1−4Ain ML1-4A-expressing HEK293T cells. (j) The effects of SMase (50 ng ml−1) treatment on SF-51-activatedIML1−4Aat neutral external pH (pH 7.4). (k) The potentiation effect of SMase was more dramatic at pH 4.6, but abolished by heat inactivation of the enzyme activity. HI-SMase: heat-inactivated SMase. For panelsdandk, data are presented as the mean±s.e.m.; thennumbers are in parentheses. Statistical comparisons were made using analysis of variance: *P<0.05. Figure 6: Regulation of TRPML1 by SMs and sphingomyelinases. ( a ) SF-51-activated whole-cell I ML1−4A was inhibited by SMs (20 μM) at low extracellular pH in ML1-4A-expressing HEK293T cells. ( b ) Insensitivity of whole-cell I ML1−Va to SMs (60 μM). ( c ) Lack of effect of ceramide (Cer, 20 μM) on whole-cell I ML1−4A . ( d ) Summary of the effects of various sphingolipids on whole-cell I ML1−4A in ML1-4A-expressing HEK293T cells. PC: phosphocholine. ( e ) SF-51-activated whole-cell I ML1−4A was potentiated by sphingosine (Sph; 5 μM) at low external pH in ML1-4A-expressing HEK293T cells. ( f ) The effects of SMase (50 ng ml −1 ) treatment on I ML1−4A at low external pH. I ML1−4A was elicited by repeated voltage ramps (−140 to + 140 mV; 400 ms) with a 4-s interval between ramps. Current amplitudes at −140 mV were used to plot the time dependence. ( g ) Representative traces of I ML1−4A before (black) and after (dark yellow) SMase treatment at two different time points, as shown in f . ( h , i ) SMase (50 ng ml −1 ) treatment alone had no (six out of seven cells; see h for an example) or small (one out of seven cells; i ) activation effect on basal whole-cell I ML1−4A in ML1-4A-expressing HEK293T cells. ( j ) The effects of SMase (50 ng ml −1 ) treatment on SF-51-activated I ML1−4A at neutral external pH (pH 7.4). ( k ) The potentiation effect of SMase was more dramatic at pH 4.6, but abolished by heat inactivation of the enzyme activity. HI-SMase: heat-inactivated SMase. For panels d and k , data are presented as the mean±s.e.m. ; the n numbers are in parentheses. Statistical comparisons were made using analysis of variance: * P <0.05. Full size image The robust inhibition of I ML1−4A by SMs, but not ceramide or phosphocholine, suggests that the activity of SMase may regulate I ML1−4A . Indeed, bath application of SMases, but not heat-inactivated enzymes, significantly potentiated SF-51-activated I ML1−4A ( Fig. 6f–k ), with the potentiation being more dramatic at acidic extracellular (luminal) pH than at neutral pH ( Fig. 6k ). SM accumulation reduces TRPML1-mediated Ca 2+ release The results presented above suggest that SM-mediated inhibition underlies NPC-mediated reduction in TRPML1-mediated lysosomal Ca 2+ release. Consistent with this, in fibroblasts derived from NPA patients, which completely lack the activity of aSMase [3] , TRPML1-mediated, but not GPN-induced, lysosomal Ca 2+ release ( Fig. 7a–c ) was significantly reduced. To further test this hypothesis, we induced lysosomal SM accumulation by incubating cells with desipramine and fluoxetine for 2–4 h, which cause proteolytic degradation of aSMase [30] , [31] . Compared with non-treated cells, TRPML1-mediated lysosomal Ca 2+ release was dramatically reduced in desipramine/fluoxetine-treated CHO cells, and the reduction was abolished in the presence of a protease inhibitor leupeptin [30] , [31] ( Fig. 7d–g ). Taken together, these results suggest that SM inhibition of TRPML1 underlies NPA- or NPC-mediated attenuation of TRPML1-mediated lysosomal Ca 2+ release. 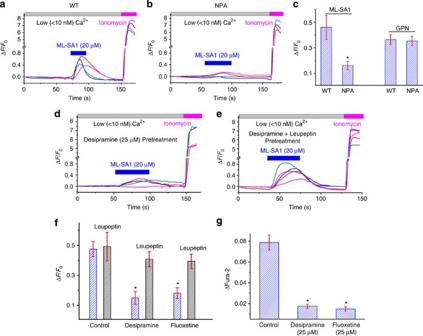Figure 7: SM accumulation in the lysosome reduces TRPML1-mediated Ca2+release. (a,b) ML-SA1-induced lysosomal Ca2+release was reduced in GCaMP3-ML1-transfected NPA fibroblasts (b) compared with WT fibroblasts (a). (c) Average ML-SA1- (20 μM) and GPN-induced (200 μM) responses in GCaMP3-ML1-transfected WT and NPA fibroblasts. (d) Desipramine (25 μM) treatment for 2–4 h reduced TRPML1-mediated lysosomal Ca2+release responses (20 μM ML-SA1) in GCaMP3-ML1-transfected CHO cells. (e) Pretreatment of a protease inhibitor leupeptin (25 μM) abolished the effects of desipramine in ML-SA1-induced GCaMP3 responses. (f) Summary of the effects of desipramine (25 μM) and fluoxetine (25 μM) treatment for 2–4 h on TRPML1-mediated lysosomal Ca2+release responses (20 μM ML-SA1) in GCaMP3-ML1-transfected CHO cells. (g) Desipramine and fluoxetine treatment for 2–4 h reduced endogenous lysosomal Ca2+release responses (measured with Fura-2 ratios; 100 μM ML-SA1) in CHO cells. For panelsc,fandg, the results were averaged for 40–100 cells from at least three independent experiments; data are presented as the mean±s.e.m. Statistical comparisons were made using analysis of variance: *P<0.05. Figure 7: SM accumulation in the lysosome reduces TRPML1-mediated Ca 2+ release. ( a , b ) ML-SA1-induced lysosomal Ca 2+ release was reduced in GCaMP3-ML1-transfected NPA fibroblasts ( b ) compared with WT fibroblasts ( a ). ( c ) Average ML-SA1- (20 μM) and GPN-induced (200 μM) responses in GCaMP3-ML1-transfected WT and NPA fibroblasts. ( d ) Desipramine (25 μM) treatment for 2–4 h reduced TRPML1-mediated lysosomal Ca 2+ release responses (20 μM ML-SA1) in GCaMP3-ML1-transfected CHO cells. ( e ) Pretreatment of a protease inhibitor leupeptin (25 μM) abolished the effects of desipramine in ML-SA1-induced GCaMP3 responses. ( f ) Summary of the effects of desipramine (25 μM) and fluoxetine (25 μM) treatment for 2–4 h on TRPML1-mediated lysosomal Ca 2+ release responses (20 μM ML-SA1) in GCaMP3-ML1-transfected CHO cells. ( g ) Desipramine and fluoxetine treatment for 2–4 h reduced endogenous lysosomal Ca 2+ release responses (measured with Fura-2 ratios; 100 μM ML-SA1) in CHO cells. For panels c , f and g , the results were averaged for 40–100 cells from at least three independent experiments; data are presented as the mean±s.e.m. Statistical comparisons were made using analysis of variance: * P <0.05. Full size image TRPML1 regulates lysosomal lipid and cholesterol trafficking Human NPC, NPA and NPB fibroblasts exhibit defects in LEL-to-Golgi trafficking of lipids and proteins [6] , [27] . Consistent with this, BODIPY-LacCer, a fluorescent analogue of lactosylceramide that is localized in the Golgi apparatus of WT cells after a pulse-chase period [32] , was predominantly localized in the LEL-like compartments of NPC1 −/− mouse macrophages ( Fig. 8a ). Owing to the established roles of PI(3,5)P 2 /TRPML1/Ca 2+ in LEL-to-Golgi lipid trafficking [15] , it is possible that the trafficking defects seen in NP cells are due to the aforementioned attenuated TRPML1-mediated lysosomal Ca 2+ release. If so, one would expect that boosting TRPML1 activity may correct the trafficking defects. Indeed, more than 60% of ML-SA1-treated NPC macrophages exhibited a Golgi-like pattern of LacCer staining, suggestive of a significant restoration in LEL-to-Golgi transport ( Fig. 8a ). In NPC1 −/− mouse macrophages and TRPML1-transfected NPC CHO cells, the puncta number of LacCer staining, that reflects the function of LEL-to-Golgi transport, was significantly reduced in the presence of ML-SA1 ( Fig. 8b and Supplementary Fig. S5 ). Collectively, these results suggest that increasing TRPML1's channel activity may restore the trafficking defects in NPC cells, and that TRPML1 deregulation is a pathogenic mechanism underlying lipid trafficking defects in NP cells. 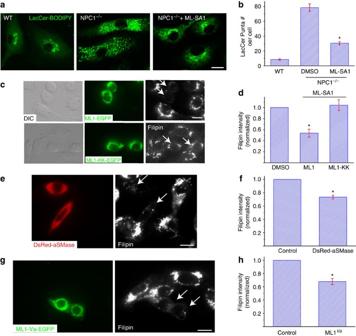Figure 8: ML-SA1 and TRPML1 overexpression rescue the trafficking defects and reduce cholesterol accumulation in NPC cells. (a) A fluorescent analogue of lactosylceramide, BODIPY-LacCer, was mainly localized in the Golgi-like structures of WT macrophages after a pulse-chase for 1 h, but accumulated in the LEL-like vesicles of NPC macrophages. ML-SA1 (10 μM) treatment of NPC1−/−macrophages for 12 h resulted in a primary Golgi-like localization for LacCer. Scale bar=10 μm. (b) ML-SA1 reduced the number of LacCer puncta in NPC1−/−macrophages. (c,d) ML-SA1 reduced unesterified cholesterol (filipin) staining in ML1, but not ML1-KK-expressing U18666A-treated WT CHO cells. Differential interference contrast (DIC) images are shown for comparison. Scale bar=10 μm. (e) Unesterified cholesterol (filipin) staining in NPC CHO cells was partially reduced in cells expressing DsRed-aSMase. (f) Average filipin staining (intensity normalized to non-transfected control cells) in DsRed-aSMase-transfected cells. (g) Unesterified cholesterol (filipin) staining in NPC CHO cells was partially reduced in cells expressing ML1-Va-EGFP (ML1Va). (h) Average filipin staining (intensity normalized to non-transfected control cells) in ML1Va-transfected cells. Scale bar=10 μm for panelsa,c,eandg. For panelsb,d,fandh, the results were averaged for multiple randomly taken micrographs from at least three independent experiments. Data are presented as the mean±s.e.m. Statistical comparisons were made using analysis of variance: *P<0.05. Figure 8: ML-SA1 and TRPML1 overexpression rescue the trafficking defects and reduce cholesterol accumulation in NPC cells. ( a ) A fluorescent analogue of lactosylceramide, BODIPY-LacCer, was mainly localized in the Golgi-like structures of WT macrophages after a pulse-chase for 1 h, but accumulated in the LEL-like vesicles of NPC macrophages. ML-SA1 (10 μM) treatment of NPC1 −/− macrophages for 12 h resulted in a primary Golgi-like localization for LacCer. Scale bar=10 μm. ( b ) ML-SA1 reduced the number of LacCer puncta in NPC1 −/− macrophages. ( c , d ) ML-SA1 reduced unesterified cholesterol (filipin) staining in ML1, but not ML1-KK-expressing U18666A-treated WT CHO cells. Differential interference contrast (DIC) images are shown for comparison. Scale bar=10 μm. ( e ) Unesterified cholesterol (filipin) staining in NPC CHO cells was partially reduced in cells expressing DsRed-aSMase. ( f ) Average filipin staining (intensity normalized to non-transfected control cells) in DsRed-aSMase-transfected cells. ( g ) Unesterified cholesterol (filipin) staining in NPC CHO cells was partially reduced in cells expressing ML1-Va-EGFP (ML1 Va ). ( h ) Average filipin staining (intensity normalized to non-transfected control cells) in ML1 Va -transfected cells. Scale bar=10 μm for panels a , c , e and g . For panels b , d , f and h , the results were averaged for multiple randomly taken micrographs from at least three independent experiments. Data are presented as the mean±s.e.m. Statistical comparisons were made using analysis of variance: * P <0.05. Full size image NPC cells accumulate cholesterol, as demonstrated by elevated filipin staining [25] . However, in U18666A-treated CHO cells, ML-SA1 induced a significant reduction in filipin staining in TRPML1, but not TRPML1-KK-transfected cells ( Fig. 8c,d ). Likewise, in TRPML1-transfected NPC CHO cells, a significant reduction of filipin staining was also seen in the presence of ML-SA1 ( Supplementary Fig. S5 ). Reduction of filipin staining was also seen in aSMase- ( Fig. 8e,f ) and TRPML1 Va -transfected NPC CHO cells ( Fig. 8g,h ). These results suggest that increased TRPML1 activity may reduce cholesterol accumulation in NPC cells. We used a lysosome-targeted GCaMP3-based Ca 2+ imaging method to demonstrate that TRPML1-mediated lysosomal Ca 2+ release, but not the lysosomal Ca 2+ store as has been reported previously [25] , is selectively compromised in NPC and NPA cells. SM, a sphingolipid that is known to accumulate in all three types of NP cells [4] , inhibits TRPML1. Pharmacologically induced SM accumulation significantly reduces TRPML1-mediated lysosomal Ca 2+ release. Conversely, increasing TRPML1's expression or activity is sufficient to correct the trafficking defects and reduce cholesterol accumulation in NPC cells. Collectively, our work provides a feedback mechanism for luminal lipids to control lipid efflux from the lysosome, as well as a pathogenic cause for the secondary lysosome storage present in many LSDs. SMs are present on the outer leaflet of the plasma membrane [33] , suggesting that SM inhibition of TRPML1 might serve as a physiological mechanism to prevent this lysosome channel from being active at the wrong subcellular location, that is, the plasma membrane. For normal cells, SMs in the lysosome would be rapidly degraded by aSMase activity [33] . In NP cells, however, SMs accumulate in the lumen and limited lysosomal membranes ( Supplementary Fig. S1 ). Although the primary storage is likely to be cholesterol, NPC cells are found to have a much lower level of aSMase activity, and a restoration of aSMase activity could revert cholesterol accumulation [34] . It is not known whether the level of SM is perturbed in other sphingolipidoses. However, rather than absolute SM levels, the relative localization (plasma membrane versus lysosome) is the factor critical for lysosomal Ca 2+ release. In addition, other offending metabolites might also inhibit TRPML1, and/or PI(3,5)P 2 -metabolizing enzymes. Thus, impaired Ca 2+ release might be a common pathogenic mechanism for many LSDs. Although TRPML1 is the dominant lysosomal TRPML channel in most cell types, in other cell types where TRPML2 and TRPML3 are more abundantly expressed [13] , our proposed SM-mediated inhibitory mechanism may also be applied to TRPML2/3, causing lysosomal trafficking defects. Finally, SM and cholesterol accumulation might also contribute to NP phenotypes via mechanisms unrelated to lysosomal trafficking and TRPMLs [3] . LEL-to-Golgi trafficking defects are seen in PI(3,5)P 2 -deficient cells [22] , ML4 fibroblasts [15] , [35] and NP fibroblasts, as well as fibroblasts from several other sphingolipid LSDs [6] , [36] . Our results suggest that reduced TRPML1-mediated lysosomal Ca 2+ release directly causes trafficking defects. We previously reported that impaired Fe 2+ homoeostasis facilitates the formation of autofluorescent lipofuscin in ML4 cells [11] . Interestingly, lipofuscin formation is also increased in NPC cells ( Supplementary Fig. S6 ). For most LSDs, impaired lysosomal degradation due to a lack of hydrolytic enzymes leads to trafficking defects and lysosome storage. However, lysosome storage can in turn affect lysosomal degradation and membrane trafficking, which results in a positive feedback loop and a vicious cycle [2] . Our work suggests a novel concept that lysosome enhancement by manipulating TRPML1 to speed membrane trafficking may break the vicious cycle, providing a novel therapeutic approach for NPs and many other LSDs. Molecular biology and biochemistry The GCaMP3-ML1 construct was made by inserting the full-length GCaMP3 sequence [24] between the HindIII and BamHI sites of a pcDNA6 plasmid that contains the mouse TRPML1 complementary DNA at the XhoI site. TRPML1-L 15 L/AA-L 577 L/AA (abbreviated as ML1-4A) and the TRPML1 non-conducting pore mutant (D471K/D472K; abbreviated as ML1-KK) were constructed using a site-directed mutagenesis kit (Qiagen). All constructs were confirmed by sequencing, and protein expression was verified by western blot. CHO, HEK293T, Cos-1 and human fibroblast cells were transiently transfected with GCaMP3-ML1 for electrophysiology, Ca 2+ imaging and confocal imaging. PCR primers used for real-time quantitative PCR analysis of TRPML expression in human fibroblasts and mouse macrophages are as follows: Human TRPML1 : F, 5′-CGGATGACACCTTCGCAGCCTAC-3′; R, 5′-ACGCATACCGGCCCAGTGACAC-3′ Human TRPML2 : F, 5′-GGTCACCACACAGCTTGTTCGT-3′; R, 5′-TGATGATACTGATTAATAGCA-3′ Human TRPML3 : F, 5′-CCAGAAATTGAAACTGAGTGTT-3′; R, 5′-ATGTTATAGTCAGAGTAAAGTC-3′ Mouse TRPML1 : F, 5′-AAACACCCCAGTGTCTCCAG-3′; R, 5′-GAATGACACCGACCCAGACT-3′ ML4 and NPC cell lines NPC (CT43; NPC1 −/− ) and WT control (RA25) CHO cells were a gift from Dr Chang TY (Dartmouth Medical School). Human skin fibroblast cells from an ML4 patient (ML1 −/− , clone GM02048), an NPC patient (NPC1 −/− , clone GM03123) and an NPA patient (clone GM00112), and non-disease control cells (ML1 +/+ / NPC1 −/− , clone GM00969) were obtained from the Coriell Institute for Medical Research (NJ, USA). Human fibroblasts were transiently transfected by electroporation (260 V, 950 μF) with 100 μg of GCaMP3-ML1 plasmid, and then used for Ca 2+ imaging experiments 24 h after electroporation. Mouse lines NPC1 KO mice (BALB/cNctr-Npc1m1N/J) and WT littermates were ordered from the Jackson Laboratories. TRPML1 knockout mice were kindly provided by Dr. Susan Slaugenhaupt (Harvard Medical School) and Dr. Jim Pickel (NIH) [37] . Animals were used under approved animal protocols and University of Michigan Institutional Animal Care Guidelines. Preparation and culture of mouse macrophages Bone marrow cells from femurs and tibias were harvested and cultured in macrophage differentiation medium (RPMI-1640 medium with 10% fetal bovine serum (FBS) and 100 U ml −1 recombinant colon stimulating factor from PeproTech, Rocky Hill, NJ, USA). After 7 days in culture at 37 °C with 5% CO 2 , the adherent cells (>95% are expected to be macrophages) were harvested for assays [38] . Mammalian whole-cell electrophysiology HEK293T, Cos-1 and CHO cells were used for the heterologous expression experiments and were transfected using Lipofectamine 2000 (Invitrogen). The pipette solution contained 147 mM Cs, 120 mM methane-sulphonate, 4 mM NaCl, 10 mM EGTA, 2 mM Na 2 -ATP, 2 mM MgCl 2 and 20 mM HEPES (pH 7.2; free [Ca 2+ ] i <10 nM). The standard extracellular bath solution (modified Tyrode's solution) contained 153 mM NaCl, 5 mM KCl, 2 mM CaCl 2 , 1 mM MgCl 2 , 20 mM HEPES and 10 mM glucose (pH 7.4). The 'Low pH Tyrode' solution contained 150 mM Na-gluconate, 5 mM KCl, 2 mM CaCl 2 , 1 mM MgCl 2 , 10 mM glucose, 10 mM HEPES and 10 mM MES (pH 4.6). All bath solutions were applied via a perfusion system to achieve a complete solution exchange within a few seconds. Data were collected using an Axopatch 2A patch clamp amplifier, Digidata 1440 and pClamp 10.0 software (Axon Instruments). Whole-cell currents were digitized at 10 kHz and filtered at 2 kHz. All experiments were conducted at room temperature (21–23 °C), and all recordings were analysed with pClamp 10.0 and Origin 8.0 (OriginLab, Northampton, MA, USA). Endolysosomal electrophysiology Endolysosomal electrophysiology was performed in isolated endolysosomes using a modified patch-clamp method [11] , [14] . Briefly, cells were treated with 1 μM vacuolin-1 for 2–5 h to increase the size of endosomes and lysosomes. Whole-endolysosome recordings were performed on isolated enlarged LELs. The bath (internal/cytoplasmic) solution contained 140 mM K-gluconate, 4 mM NaCl, 1 mM EGTA, 2 mM Na 2 -ATP, 2 mM MgCl 2 , 0.39 mM CaCl 2 , 0.2 mM GTP and 10 mM HEPES (pH adjusted with KOH to 7.2; free [Ca 2+ ] i ~100 nM based on the Maxchelator software ( http://maxchelator.stanford.edu/ )). The pipette (luminal) solution consisted of a 'Low pH Tyrode's solution' with 145 mM NaCl, 5 mM KCl, 2 mM CaCl 2 , 1 mM MgCl 2 , 10 mM HEPES, 10 mM MES and 10 mM glucose (pH 4.6). Fura-2 Ca 2+ imaging Cells were loaded with 5 μM Fura-2 AM in the culture medium at 37 °C for 60 min. Fluorescence was recorded at different excitation wavelengths using an EasyRatioPro system (PTI). Fura-2 ratios ( F 340 / F 380 ) were used to monitor changes in intracellular [Ca 2+ ] upon stimulation. GPN (200–400 μM, a lysosome-disrupting agent) and Baf-A1 (500 nM, a V-ATPase inhibitor) were used as positive controls to induce Ca 2+ release from lysosome and acidic stores, respectively [39] . Ionomycin (1 μM) was added at the conclusion of all experiments to induce a maximal response for comparison. For endogenous lysosomal Ca 2+ release measurement, Ca 2+ imaging was carried out within 0.5–3 h after plating and when cells still exhibited a round morphology. GCaMP3 Ca 2+ imaging At 18–24 h after transfection with GCaMP3-ML1, CHO or human fibroblast cells were trypsinized and plated onto glass coverslips. Most experiments were carried out within 0.5–3 h after plating when cells still exhibited a round morphology. The fluorescence intensity at 470 nm (F 470 ) was monitored using the EasyRatioPro system. Lysosomal Ca 2+ release was measured under a 'low' external Ca 2+ solution, which contained 145 mM NaCl, 5 mM KCl, 3 mM MgCl 2 , 10 mM glucose, 1 mM EGTA and 20 mM HEPES (pH 7.4). Ca 2+ concentration in the nominally free Ca 2+ solution is estimated to be 1–10 μM. With 1 mM EGTA, the free Ca 2+ concentration is estimated to be <10 nM based on the Maxchelator software ( http://maxchelator.stanford.edu/ ). LacCer-BODIPY trafficking Cells for the Lactosylceramide (LacCer)-BODIPY uptake experiment were grown on glass coverslips and incubated with 5 μM bovine serum albumin-complexed LacCer in 'Tyrode' solution for 45 min at room temperature. Cells were then washed twice with PBS and incubated with normal DMEM/F12 medium containing 10% FBS at 37 °C for 1 h. For the correction experiments, NPC1 −/− macrophages were pretreated with ML-SA1 (10 μM) for 12 h, and chased in the presence of ML-SA1 (10 μM). Images were taken using a Leica (TCS SP5) confocal microscope. Filipin staining Cells were fixed in 3% paraformaldehyde for 1 h, washed twice with PBS and then incubated with 1.5 mg ml −1 glycine in PBS for 10 min. Cells were then stained for 2 h with 0.05 mg ml −1 filipin [25] in PBS supplemented with 10% FBS. All procedures were conducted at room temperature. Images were taken using a fluorescence microscope with a UV filter. The lysosome-like storage organelle filipin intensity was calculated based on low- and high-threshold intensities in the image [34] . Lysenin staining Cells were fixed with 4% Paraformaldehyde (PFA) for 20 min, blocked with 1% bovine serum albumin in Phosphate Buffer Saline with 0.1%(v/v) Tween-20 (PBST) for 2 h and then incubated with lysenin (0.1 μg ml −1 , Peptides International) for 20 h at 4 °C. The cells were then incubated with anti-lysenin antibody (Peptides International) for 1 h, followed by Alexa Fluor 488 anti-rabbit (Invitrogen) for 45 min. Images were taken using a Leica confocal microscope. Reagents Sphingomyelins (Sigma) were dissolved in 'Tyrode' or 'Low pH Tyrode' solutions by sonication. β-cyclodextrin, filipin and fluoxetine were obtained from Sigma; desipramine was purchased from Santa Cruz; C6-ceramide was obtained from Matreya, LLC; sphingomyelinase was obtained from MP Biomedicals; SF-51 and ML-SA1 were purchased from Princeton BioMolecular Research Inc; PI(3,5)P 2 was purchased from Echelon; U18666A was purchased from Enzo; LacCer-BODIPY was purchased from Invitrogen, and lysenin and anti-lysenin antibody were purchased from Peptides International. Data analysis Data are presented as the mean±s.e.m.. Statistical comparisons were made using analysis of variance. A P -value <0.05 was considered statistically significant. How to cite this article: Shen, D. et al . Lipid storage disorders block lysosomal trafficking by inhibiting a TRP channel and lysosomal calcium release. Nat. Commun. 3:731 doi: 10.1038/ncomms1735 (2012).